Fast coherent manipulation of three-electron states in a double quantum dot An important goal in the manipulation of quantum systems is the achievement of many coherent oscillations within the characteristic dephasing time T 2 * . Most manipulations of electron spins in quantum dots have focused on the construction and control of two-state quantum systems, or qubits, in which each quantum dot is occupied by a single electron. Here we perform quantum manipulations on a system with three electrons per double quantum dot. We demonstrate that tailored pulse sequences can be used to induce coherent rotations between three-electron quantum states. Certain pulse sequences yield coherent oscillations fast enough that more than 100 oscillations are visible within a T 2 * time. The minimum oscillation frequency we observe is faster than 5 GHz. The presence of the third electron enables very fast rotations to all possible states, in contrast to the case when only two electrons are used, in which some rotations are slow. Electrons in semiconductor quantum dots are promising candidates for use in quantum computing, because of the potential of this platform to enable coherent quantum control on large numbers of qubits [1] . Much recent progress has led to demonstrations of both spin- and charge-based qubits in both GaAs and Si (refs 2 , 3 , 4 , 5 , 6 , 7 , 8 , 9 , 10 , 11 , 12 ). A necessary requirement for quantum information processing is the ability to manipulate quantum states in times that are much shorter than the decoherence time (ref. 13 ). Charge qubits can be manipulated quickly but have relatively short coherence times, whereas spin qubits have long coherence times but long manipulation times. The tendency of the speed of manipulation to be correlated with the rate of decoherence is not surprising, because both depend on the coupling of the qubit to external degrees of freedom—designed and wanted for manipulation, and extraneous and unwanted for decoherence. Shi et al . [14] and Koh et al . [15] , which describe a quantum dot hybrid qubit, present theoretical arguments that a system with more degrees of freedom, specifically three electrons in two quantum dots, can overcome this tendency. Two of the states can form a qubit with spin character that has a long coherence time. By accessing a third state via a charge transition, fast operations can be performed and then the qubit can be converted back into a spin-like qubit with long coherence time. Such a strategy requires that one can systematically and accurately control transitions between several different quantum states of a system with three electrons in two quantum dots. This Article presents experiments that demonstrate the ability to tailor transitions between quantum states of three electrons in two quantum dots (see Methods for details of device fabrication). Four states are important in this work, the ground |0 and first excited state |1 of the dot in the (2,1) charge occupation, and the corresponding ground |2 and first excited state |3 of the dot in the (1,2) charge occupation. The qubits are manipulated by pulsing a voltage that changes the detuning ε , which is the energy difference between the two dots. By applying appropriate sequences of voltage pulses, oscillations between different pairs of quantum levels can be induced. Because oscillations with periods much shorter than the rise times of the applied pulses can be excited, and because quantum oscillations between some pairs of the states are quite insensitive to the dominant dephasing mechanism, which is fluctuations in the value of the detuning [16] , many (over a hundred) oscillations can be observed within one coherence time. The consistency of our interpretation of the data in terms of coherent quantum oscillations between different energy levels is demonstrated by the agreement between the data, which were all taken with one tuning of the dot, and the simulations shown, which were all performed with one set of values for the system parameters. 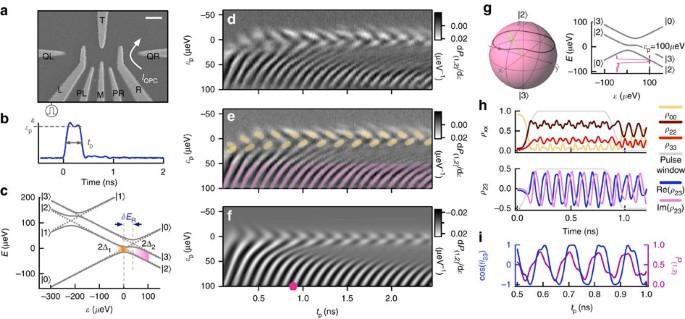Figure 1: Measurement of quantum oscillations between three quantum states of three electrons in two quantum dots. (a) Scanning electron micrograph of a device identical to the one used in the experiment. The scale bar is 200 nm in length. The currentIQPCthrough the quantum point contact (QPC) is used for charge sensing through a measurement of its transconductanceGL=∂IQPC/∂VL, whereVLis the voltage on gate L. (b) A typical pulse trace from the output of the Agilent 81134A pulse generator, with pulse widthtp. (c) Diagram of energy levels of the system versus detuningε. The (2,1) state |0anticrosses with the (1,2) states |2and |3with tunnel couplings Δ1and Δ2. The two anticrossings are separated by an energy of δER, which is the singlet-triplet energy splitting in the right dot. Colours correspond to features in the data described in (e). (d) Measurement of the transconductance through the QPC, which reflects changes in the charge occupation of the double dot, as a function of pulse durationtpand detuning of the pulse tipεp. (e) Data from (d) in which different oscillation frequencies are highlighted in colour. The orange features at small detuning with frequency ~5 GHz are charge qubit oscillations8,9,10,17,18between the states |0and |2. The pink features with frequency ~9 GHz that occur at larger values of the detuning reflect phase winding between states |2and |3. (f) Results of the calculated quantum dynamics (see Methods for details) of a system with energy separation between |2and |3of δER=9.2 GHz and tunnel couplings Δ1=2.62 GHz and Δ2=3.5 GHz, including low-frequency noise in detuning as in Peterssonet al.8(g) Left: Bloch sphere of the projection of the wavefunction onto the |2, |3subspace with the trajectory of the state vector during theεp-portion of the pulse mapped out for the case ofεp=100 μeV. Right: the relative position of the pulse and the energy diagram for the data point labelled with pink pentagon (εp=100 μeV,tp=800 ps) in (f). (h) Top: computed time evolution of the diagonal elements of the density matrix during the pulse for the data point labelled with pink pentagon in (f). The rising edge of the pulse increases the population of states |2and |3to 70 and 23%, respectively. Bottom: Time evolution of off-diagonal terms in the density matrix for the data point labelled with pink pentagon in (f). Relative phase oscillations between the two states during theεp-portion of the pulse are clearly visible. (i) The relative phaseθ23of states |2and |3, taken at the half point of the falling edge of the pulse, as a function of pulse width and the probability of measuring (1,2) charge occupation as a function of pulse width. The two curves are well correlated with each other, indicating the phase oscillation information during the pulse is mapped to charge probability by the falling edge of the pulse. Coherent oscillations from a square gate voltage pulse Figure 1a shows a device identical to the gated Si/SiGe quantum dot we study here. The simple pulse sequence shown in Fig. 1b has been used in previous work to investigate quantum oscillations between states of a charge qubit [8] , [9] , [10] , [17] , [18] . Here we demonstrate that oscillations both between states |0 and |2 and between states |2 and |3 can be established and measured by application of a gate voltage pulse with this shape. Figure 1c shows an energy level diagram where the energy splittings are determined by matching simulations discussed below to the data we present; we note that the energy splittings in the left and right dot differ, probably because of the role of valley states in Si quantum dots [19] . In this pulsed gate voltage experiment, the detuning voltage starts at a negative base value, where state |0 is favored energetically, and then it is pulsed to more positive detuning, close to the |0 -|2 and |0 -|3 anticrossings. After a short time (typically of order 1–10 ns), the pulse ends and the detuning returns to its base value. Figure 1d shows the resulting transconductance of the quantum point contact (QPC) indicated on Figure 1a , which is sensitive to changes in the time-averaged charge occupation of the dot. If the electron is in one of the (1,2) states, |2 or |3 , at the end of the pulse, it remains in that state until it decays inelastically back to a (2,1) state, which takes ~18 ns (ref. 10 ). Thus, the average charge distribution in the dot reflects the occupation of the dot just after the end of the pulse. Two different types of oscillations are observed and are highlighted in orange and pink in Fig. 1e : the former occur near the anticrossing between |0 and |2 and have a frequency that depends strongly on detuning. The latter arise for ε p more positive than the former; they have a frequency that is nearly independent of detuning and that reflects the energy difference between states |2 and |3 , as we show below. Figure 1: Measurement of quantum oscillations between three quantum states of three electrons in two quantum dots. ( a ) Scanning electron micrograph of a device identical to the one used in the experiment. The scale bar is 200 nm in length. The current I QPC through the quantum point contact (QPC) is used for charge sensing through a measurement of its transconductance G L = ∂ I QPC / ∂ V L , where V L is the voltage on gate L. ( b ) A typical pulse trace from the output of the Agilent 81134A pulse generator, with pulse width t p . ( c ) Diagram of energy levels of the system versus detuning ε . The (2,1) state |0 anticrosses with the (1,2) states |2 and |3 with tunnel couplings Δ 1 and Δ 2 . The two anticrossings are separated by an energy of δ E R , which is the singlet-triplet energy splitting in the right dot. Colours correspond to features in the data described in ( e ). ( d ) Measurement of the transconductance through the QPC, which reflects changes in the charge occupation of the double dot, as a function of pulse duration t p and detuning of the pulse tip ε p . ( e ) Data from ( d ) in which different oscillation frequencies are highlighted in colour. The orange features at small detuning with frequency ~5 GHz are charge qubit oscillations [8] , [9] , [10] , [17] , [18] between the states |0 and |2 . The pink features with frequency ~9 GHz that occur at larger values of the detuning reflect phase winding between states |2 and |3 . ( f ) Results of the calculated quantum dynamics (see Methods for details) of a system with energy separation between |2 and |3 of δ E R =9.2 GHz and tunnel couplings Δ 1 =2.62 GHz and Δ 2 =3.5 GHz, including low-frequency noise in detuning as in Petersson et al . [8] ( g ) Left: Bloch sphere of the projection of the wavefunction onto the |2 , |3 subspace with the trajectory of the state vector during the ε p -portion of the pulse mapped out for the case of ε p =100 μeV. Right: the relative position of the pulse and the energy diagram for the data point labelled with pink pentagon ( ε p =100 μeV, t p =800 ps) in ( f ). ( h ) Top: computed time evolution of the diagonal elements of the density matrix during the pulse for the data point labelled with pink pentagon in ( f ). The rising edge of the pulse increases the population of states |2 and |3 to 70 and 23%, respectively. Bottom: Time evolution of off-diagonal terms in the density matrix for the data point labelled with pink pentagon in ( f ). Relative phase oscillations between the two states during the ε p -portion of the pulse are clearly visible. ( i ) The relative phase θ 23 of states |2 and |3 , taken at the half point of the falling edge of the pulse, as a function of pulse width and the probability of measuring (1,2) charge occupation as a function of pulse width. The two curves are well correlated with each other, indicating the phase oscillation information during the pulse is mapped to charge probability by the falling edge of the pulse. Full size image Simulations To gain insight into the two different oscillation frequencies shown in Fig. 1d,e , we report in Fig. 1f–i numerical simulations (see Methods for details) of the dynamics of a system with the energy spectrum shown in Fig. 2a , with low-frequency detuning noise incorporated as in Petersson et al . [8] Figure 1f shows the result of the simulation, which is in good agreement with the data. When ε p ≈0, the oscillations (highlighted with orange in Fig. 1e ) are between the states |0 and |2 , the ground states of the (2,1) and (1,2) charge occupations. The ‘sideways-v’, criss-cross pattern of the oscillations in this regime is characteristic of lock-in measurement of charge qubits [8] , [9] , [10] , [18] ; it arises because the oscillation frequency depends strongly on ε p , with a minimum frequency of 2Δ 1 at ε p =0. At larger values of ε p , oscillations at a different frequency appear (highlighted by the nearly parallel pink lines near the bottom of Fig. 1e ). These oscillations have a different period (~100 ps) that depends only weakly on ε p ; they are well-described by the simulation of Fig. 1f , and their frequency is set by the energy difference between the states |2 and |3 . As is clear from the full time evolution of each relevant state, which is plotted in Fig. 1h , at this detuning the rising edge of the pulse transfers the large majority of the weight in the wavefunction into states |2 and |3 , leaving very little occupation of |0 . 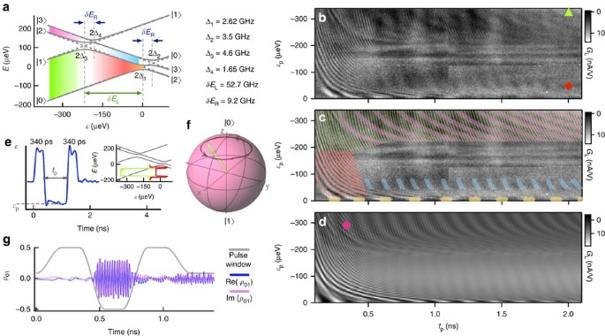Figure 2: Coherent oscillations between several pairs of states can be observed with a simple multilevel gate voltage pulse. (a) Diagram of relevant energy levels of the electrons in the double quantum dot. The oscillations highlighted in the measurements shown in panel (c) correspond to the transitions between levels denoted by the appropriately coloured regions in this diagram. The parameters used in the simulation are also listed. (b) Measured transconductance through the charge sensing QPC, which reflects changes in the time-averaged charge state of the double quantum dot as a function of the pulse detuningεpand of the pulse durationtp, with all other parameters held fixed, in the presence of the pulse sequence in (e). Coherent oscillations between different pairs of charge states are reflected in the oscillation of the time-averaged charge occupation in the dot as a function oftpat different values of the detuning. (c) Same as (b) with the different frequencies highlighted by differently coloured lines. The oscillations highlighted here correspond to the transitions between levels denoted by the corresponding coloured regions in (a). (d) Results of numerical simulation of the system with parameters listed in (a), in the presence the pulse sequence in (e). The pulse rise time used is 118 ps. (e) A typical pulse trace for this experiment. Inset: the relative position of the pulses with respect to the energy levels for the data points labelled by the green triangle and red diamond in (b). (f) Projection onto the Bloch sphere for the states |0and |1, with the trajectory of the state vector during theεp-portion of the pulse mapped out atεp=−291 μeV. (g) Computed time evolution of the coupling term between states |0and |1for the data point labelled with the pink pentagon in (d). Relative phase oscillations between the two states during theεp-portion of the pulse are clearly visible. An approximate quantum wavefunction during the ε p -portion of the pulse is thus given by Figure 2: Coherent oscillations between several pairs of states can be observed with a simple multilevel gate voltage pulse. ( a ) Diagram of relevant energy levels of the electrons in the double quantum dot. The oscillations highlighted in the measurements shown in panel ( c ) correspond to the transitions between levels denoted by the appropriately coloured regions in this diagram. The parameters used in the simulation are also listed. ( b ) Measured transconductance through the charge sensing QPC, which reflects changes in the time-averaged charge state of the double quantum dot as a function of the pulse detuning ε p and of the pulse duration t p , with all other parameters held fixed, in the presence of the pulse sequence in ( e ). Coherent oscillations between different pairs of charge states are reflected in the oscillation of the time-averaged charge occupation in the dot as a function of t p at different values of the detuning. ( c ) Same as ( b ) with the different frequencies highlighted by differently coloured lines. The oscillations highlighted here correspond to the transitions between levels denoted by the corresponding coloured regions in ( a ). ( d ) Results of numerical simulation of the system with parameters listed in ( a ), in the presence the pulse sequence in ( e ). The pulse rise time used is 118 ps. ( e ) A typical pulse trace for this experiment. Inset: the relative position of the pulses with respect to the energy levels for the data points labelled by the green triangle and red diamond in ( b ). ( f ) Projection onto the Bloch sphere for the states |0 and |1 , with the trajectory of the state vector during the ε p -portion of the pulse mapped out at ε p =−291 μeV. ( g ) Computed time evolution of the coupling term between states |0 and |1 for the data point labelled with the pink pentagon in ( d ). Relative phase oscillations between the two states during the ε p -portion of the pulse are clearly visible. Full size image with ( t ) a global phase that does not affect measurable quantities. While the charge sensing measurement does not distinguish between states |2 and |3 , the oscillations are visible in this experiment because the two contributions interfere when the pulse ends and the detuning passes back through the two anticrossings shown in Fig. 1c , between |0 and |2 as well as |0 and |3 , so that the occupation of the (1,2) charge state after the pulse has ended oscillates with angular frequency δ E R / ħ . This relationship between the phase difference between the amplitudes in |2 and |3 and the probability of occupying the (1,2) charge state P (12) is illustrated in Fig. 1i . The physical mechanism giving rise to the ability to measure oscillations between two states with the same charge distribution via a time-averaged charge measurement is closely related to Landau-Stückelberg-Zener oscillations [20] , [21] , [22] , so we will refer to these oscillations as LSZ oscillations. For the LSZ oscillations, the coherence time T 2 *=3.7 ns, extracted from the oscillation decay at times longer than those shown in Fig. 1d . The ratio of the coherence time to the oscillation period of the LSZ oscillations between |2 and |3 is much larger than that of the charge qubit oscillations between |0 and |2 , for two reasons. First, the frequency of the LSZ oscillations is not limited by the pulse rise time; the oscillation frequency is determined by the energy difference δ E R between state |2 and |3 ; whether a particular pulse rise time results in a state in which |2 and |3 both have substantial occupation is determined by the value of the tunnel couplings Δ 1 and Δ 2 . Second, the energy difference δ E R depends only weakly on detuning [23] , so the LSZ oscillations are less susceptible to the dominant source of decoherence [8] , [9] , [24] , fluctuations in the detuning, than are oscillations between energy levels with different dependences on the detuning, such as the levels |0 and |2 used for a standard charge qubit. Coherent oscillations from a multilevel pulse We now show that more complex pulse sequences can establish oscillations between different pairs of states in the system, including between states that are both excited states of the system at all values of the detuning accessed during the sequence. Figure 2b shows the measured transconductance of the QPC charge sensor during application of a three-level pulse; Fig. 2c shows the same data with colour added for discussion; and Fig. 2d shows the corresponding simulations. The three-level pulse is shown in Fig. 2e for one particular amplitude ε p . Five distinct oscillation patterns can be identified, as shown with the colour overlay in Fig. 2c , and with corresponding colours in Fig. 2a . The numerical simulation of Fig. 2d , which uses the same parameters as the simulation in Fig. 1f , shows that the oscillation frequencies in the data correspond to energy level differences between specific pairs of quantum states. That mapping is shown in Fig. 2a , and the validity of our model is demonstrated by the accuracy of Fig. 2d . The colour overlays in Fig. 2a,c show that, even with a single, relatively simple pulse pattern, quantum superpositions and oscillations can be observed between nearly all possible pairs of states. The relative weight of each of these oscillations, which reflects the relative weight of the wavefunction in each rung in the ladder of energy eigenstates, is determined by the pulse rise time, the pulse detuning and the tunnel couplings that determine the size of the anticrossings between the three-electron states. The measurements described above have a close relationship to the quantum dot hybrid qubit [14] , [15] . One important reason for manipulating quantum states is to perform quantum information processing. For this application, one needs to create quantum gates, which are unitary transformations. If one defines a qubit as two states and , then to qualify as a gate, a process that transforms must transform either or . Koh et al . [15] presents pulse sequences that, when applied to a double quantum dot with three electrons, yield any prescribed rotation on the Bloch sphere of a qubit with basis states , , where |0 and |1 are two of the states we study here. A π rotation that sends |0 →|1 can be implemented by performing successive π rotations at the two successive anticrossings marked Δ 1 and Δ 3 in Fig. 2a . Here we can understand the oscillations highlighted green in Fig. 2c in the language of the hybrid qubit. The first 340 ps pulse in Fig. 2e rotates significant weight of the wavefunction from |0 into state |2 , which would be called an auxilliary state in a (2,1) hybrid qubit. The second, variable section of the pulse pushes the double dot to deep negative detuning, with very different effects on the fraction of the wavefunction in states |0 and |2 . State |0 simply slides to lower energy in the detuning plot shown in Fig. 2a . State |2 , in contrast, moves to higher energy, where it anticrosses with |1 . This anticrossing, governed by tunnel coupling Δ 3 , is large enough that the pulse is largely adiabatic and therefore the majority of the weight in |2 follows the lower branch to state |1 , whose dependence of energy on detuning is nearly the same as |0 , setting up a superposition whose phase difference is relatively immune to noise in detuning. Thus, this first part of the pulse is a variation on the pulsed gate previously proposed in Koh et al . [15] , and it corresponds to an -rotation from |0 to |1 . The second 340 ps pulse in Fig. 2e reverses this process, bringing the system quasi-adiabatically back through anticrossing Δ 3 , and driving a second rotation at the Δ 1 anticrossing. This pulse thus enables observation of interference as a function of the evolved phase difference between states |0 and |1 , as visible in the simulation results reported in Fig. 2f,g . Thus, the oscillations shown in green reflect a controlled phase evolution between states |0 and |1 , a -rotation for the hybrid qubit. Together the - and -rotations demonstrate fast, all electrical two-axis control, a key ingredient in constructing a pulse-gated quantum dot hybrid qubit [15] . We have demonstrated that high-speed voltage pulses can be used to control coherent quantum oscillations between different pairs of states in a semiconducting double quantum dot with three electrons. By implementing appropriate combinations of voltage pulses, oscillations between different pairs of levels as well as sequential operations can be achieved. Transitions between some pairs of levels can be induced that have over a hundred oscillations within a coherence time. All of the observed rotations and oscillations have frequencies in excess of 5 GHz. Fast rotation rates and long coherence alone are of course not sufficient to create a high-quality single qubit. An important future step to make these three-electron states useful for quantum computing is the characterization and achievement of high-fidelity rotations. The results presented here provide strong evidence that coherent, fast oscillations can be initiated and controlled between multiple levels of three electrons in a double quantum dot. Experiment The experiments are performed on a double quantum dot fabricated in a Si/SiGe heterostructure, as described in Shi et al . [10] , Thalakulam et al . [25] , and Simmons et al . [26] ; a scanning electron microscope image of an identical device is shown in Fig. 1a . By adjusting the gate voltages appropriately, we tune the dot occupation so that the valence charge occupation of the double dot is (2,1) or (1,2), where the first (second) number is the charge occupation in the left (right) dot, as confirmed by magnetospectroscopy measurements [23] . Either or both dots may contain a closed shell beneath the valence electrons; if present, such shells do not appear to play a role in the work we report. We note that the energy spacing between the ground and first excited states in the left and right dots is quite different; this difference is not unusual in Si quantum dots and likely arises because of the valley degree of freedom [27] . Theory Numerical simulations of the experiment were performed based on the energy level diagram in Fig. 2a using the pulse rise time of 118 ps. We model the dynamical evolution of the density matrix ρ of the system as a function of detuning ε and pulse duration t p using a master equation [28] : The Hamiltonian, written in the basis of position eigenstates, is The (1,2) charge occupation probability is extracted at the end of the pulse and is averaged over 2 ns in the measurement stage of the pulse. Using this number as an initial value, P (1,2) is then allowed to relax exponentially to the ground state (2,1) occupation with a relaxation time T 1 , during the measurement phase. Finally, the simulated charge occupation is determined by averaging the charge state for the entire 33 ns pulse period. Low-frequency fluctuations in the detuning ε are incorporated following Petersson et al . [8] , by performing a convolution of the results at each ε with a Gaussian in ε of width σ ε =5 μeV. The best fit to the data is found with a charge T 1 =18 ns. How to cite this article: Shi, Z. et al . Fast coherent manipulation of three-electron states in a double quantum dot. Nat. Commun. 5:3020 doi: 10.1038/ncomms4020 (2014).